RETRACTED ARTICLE: RNA m6A methylation regulates the epithelial mesenchymal transition of cancer cells and translation of Snail N6 -Methyladenosine (m 6 A) modification has been implicated in the progression of several cancers. We reveal that during epithelial-mesenchymal transition (EMT), one important step for cancer cell metastasis, m 6 A modification of mRNAs increases in cancer cells. Deletion of methyltransferase-like 3 (METTL3) down-regulates m 6 A, impairs the migration, invasion and EMT of cancer cells both in vitro and in vivo. m 6 A-sequencing and functional studies confirm that Snail, a key transcription factor of EMT, is involved in m 6 A-regulated EMT. m 6 A in Snail CDS, but not 3’UTR, triggers polysome-mediated translation of Snail mRNA in cancer cells. Loss and gain functional studies confirm that YTHDF1 mediates m 6 A-increased translation of Snail mRNA. Moreover, the upregulation of METTL3 and YTHDF1 act as adverse prognosis factors for overall survival (OS) rate of liver cancer patients. Our study highlights the critical roles of m 6 A on regulation of EMT in cancer cells and translation of Snail during this process. Among the more than 100 modifications in mRNA, N 6 -methyladenosine (m 6 A) has been identified since the 1970s [1] . m 6 A modification is the most abundant in eukaryotic mRNAs [2] , while thousands of RNA transcripts contain m 6 A modifications with unique distribution patterns as well [3] . An important report by Jia et al. [4] identified the first RNA demethylase, fat mass and obesity-associated protein (FTO),  revealing that RNA modification is reversible. Since then, the study of dynamic of m 6 A modification has greatly expanded [5] , [6] , [7] , [8] , [9] . Methyltransferase-like 3 (METTL3), METTL14, and Wilm’s tumor-1-associated protein (WTAP) have been proved to act as m 6 A methyltransferases (“writers”) in mammalian cells [10] , [11] . m 6 A-binding proteins with YTH domain, including cytoplasmic protein YTHDF1, YTHDF2, YTHDF3, and nuclear protein YTHDC1, have been identified to be the “readers” of m 6 A and modulate mRNA stability and translation to mediate downstream effects [6] , [7] , [12] , [13] . Studies on biological functions of m 6 A modification in mRNA have arisen in recent years [14] . It has been reported that m 6 A modification is involved in various biological processes, including heat-shock response [12] , ultraviolet-induced DNA damage response [15] , maternal mRNA clearance [5] , neuronal functions and sex determination [16] , cortical neurogenesis [17] , haematopoietic stem and progenitor cell specification [18] , and T-cell homeostasis [19] . Although, m 6 A modification has been associated with tumorigenesis and progression of cancer cells, the molecular mechanisms involved have not been described yet. Recently, FTO has been shown to be an oncogenic factor in acute myeloid leukemia, which functions as N6 -methyladenosine RNA demethylase [20] . Inhibition of FTO suppresses tumor progression and prolongs lifespan of glioblastoma stem cells (GSC)-grafted mice substantially [21] . Also, FTO inhibition exerts a broad anti-leukemic activity in vitro and in vivo [22] . Another identified m 6 A demethylase, ALKBH5, maintains tumorigenicity of glioblastoma stem-like cells by sustaining FOXM1 expression and cell proliferation program [23] . ALKBH5-mediated m 6 A-demethylation of NANOG mRNA is involved in hypoxia-induced breast cancer stem cell phenotype [24] . Together, these results suggest that m 6 A modification found in mRNA may regulate the progression of cancer development. The metastasis of cancer cells is responsible for more than 90% of cancer-associated mortality [25] , and epithelial–mesenchymal transition (EMT) is considered to be an important step for cancer cell metastasis. During EMT process, epithelial cells lose polarity and gain invasive properties to become mesenchymal stem cells [26] . Loss of E-cadherin (E-Cad, encoded by the CDH1 gene) has been considered as the most fundamental event in EMT program [27] . Repression of E-Cad expression, by EMT-inducing transcription factors (EMT-TFs), such as Snail, Slug, Twist, and Zeb, results in promotion of metastasis in cancer cells [28] . Snail (encoded by SNAI1), acts as a key transcriptional repressor of E-cad expression in EMT, confers tumor cells with cancer stem cell-like traits and promotes drug resistance, tumor recurrence, and metastasis [29] . Recent evidences indicated that epigenetic modifications regulate progression of EMT and cancer development [30] . Snail recruits chromatin modifiers, such as lysine-specific demethylase 1 (LSD1) [31] and Suv39H1 histone methyltransferases [32] , and triggers both transient and long-lasting chromatin changes of CDH1 promoter [33] . However, the precise role of RNA epigenetic factors on progression of EMT has not been reported yet. This study revealed a significant increase of m 6 A levels in cancer cells undergoing EMT. However, METTL3-deleted cells were less inducible for EMT. The m 6 A-seq and m 6 A-RIP-qPCR results showed that EMT induced elevation of m 6 A in CDS of SNAI1, the key inducer of EMT, and promoted YTHDF1-mediated Snail translation. Our study revealed that m 6 A regulated the progression of EMT and translation of Snail. EMT in cancer cells is regulated by m 6 A levels of mRNAs Although EMT can be induced by various extracellular ligands, TGF-β has been considered as the major inducer of this transdifferentiation process of cancer cells [34] . We treated HeLa and HepG2 cells with 10 ng/ml TGF-β for 3 days. Both TGF-β treated HeLa and HepG2 cells became scattered and adopted the fibroblast-like morphology described for mesenchymal cells (Supplementary Fig. 1A ). TGF-β treatments significantly increased wound healing (Supplementary Fig. 1B ) and in vitro invasion ability (Supplementary Fig. 1C ) of both HeLa and HepG2 cells. Moreover, upregulation of FN1 (fibronectin) and MMP2 mRNA and downregulation of CDH1 (E-Cad) mRNA were observed by qRT-PCR (Supplementary Fig. 1D). These TGF-β-induced changes in expression of EMT markers were further confirmed by western blot analysis (Supplementary Fig. 1E ). All these data indicated that cancer cells, treated with TGF-β, were undergoing EMT processes. We then investigated the variations of m 6 A levels in mRNAs of cancer cells undergoing EMT. By using LC-MS/MS, we identified that the m 6 A levels of mRNAs isolated from HeLa and HepG2 cells, treated with TGF-β, were statistically ( p < 0.05, t test) more abundant than that of their corresponding control cells (Fig. 1a ). The m 6 A/A levels of mRNA from HeLa and HepG2 cells undergoing EMT increased 20.0% and 14.9%, respectively. This was further confirmed by the results obtained in dot-blot analysis (Supplementary Fig. 2A ). Similarly, LC/MS/MS showed that m 6 A levels of mRNAs isolated from Huh7 and A549 cells, treated with TGF-β, were statistically ( p < 0.05, t test) more abundant than that of their corresponding control cells (Supplementary Fig. 2B ). Collectively, these data showed that cancer cells undergoing EMT increased m 6 A levels of mRNAs. Fig. 1 EMT in cancer cells is regulated by m 6 A levels of mRNAs. a HeLa and HepG2 cells were treated with or without 10 ng/ml TGF-β for 3 days, the m 6 A/A ratio of the total mRNA were determined by LC–MS/MS. b Wound healing of wild-type (control) or Mettl3 Mut/− cells was recorded ( left ) and quantitatively analyzed ( right ). c Wild-type or Mettl3 Mut/− cells were allowed to invade for 24 h and tested by CytoSelect™ 24-well Cell Invasion assay kits (8 µm, colorimetric format); d, e mRNA ( d ) and protein ( e ) expressions of MMP2, FN, and E-Cad in wild-type and Mettl3 Mut/− HeLa cells were measured by qRT-PCR and western blot analysis, respectively. f HeLa cells were transfected with pcDNA/ALKBH5 or a vector control for 48 h, protein expression was determined by western blot analysis (left) and quantitatively analyzed (right). g Wild-type or Mettl3 Mut/− cells were treated with or without 10 ng/ml TGF-β for 3 days, protein expression was determined by western blot analysis (left) and quantitatively analyzed (right). h The expression of METTL3 in liver cancer and its matched adjacent normal tissues of 50 patients from TCGA database. i Correlation between METTL3 and CDH1 in liver cancer patients ( n = 364) from TCGA database. j HeLa cells were pretreated with or without Smad2/3 inhibitor SB431542 (10 μM) and then further treated with 10 ng/ml TGF-β for 3 days, the m 6 A/A ratio of the total mRNA were determined by LC–MS/MS. Data are presented as means ± SD from three independent experiments. * p < 0.05, ** p < 0.01, NS, no significant, by Student’s t test. Red bar = 200 μm Full size image To characterize the roles of m 6 A in EMT process, we used Mettl3 Mut/− HeLa cells (Supplementary Fig. 2C ) generated in our previous study [35] by using the CRISPR/Cas9 editing system according to the published protocol [35] , [36] . The results showed that Mettl3 Mut/− cells had significantly lower levels of m 6 A than wild-type cells (Supplementary Fig. 2D ), which also confirmed the roles of METTL3 as m 6 A “writer” of mRNA. We evaluated the EMT-related characteristics of Mettl3 Mut/− cells. The results showed that both wound healing (Fig. 1b ) and in vitro invasion abilities (Fig. 1c ) of Mettl3 Mut/− HeLa cells were suppressed when compared with wild-type cells. Similarly, sh-Mettl3 or si-Mettl3-mediated knockdown of METTL3 suppressed the in vitro invasion of Huh7 and HepG2 cells, respectively (Supplementary Fig. 2E ). The mRNA and protein levels of both MMP2 and FN were downregulated, while E-Cad mRNA and protein levels were upregulated in Mettl3 Mut/− HeLa cells (Fig. 1d, e ). In addition, western blot analysis confirmed that METTL3 knockdown decreased MMP2 and FN, while increased E-Cad, in both Huh7 and HepG2 cells (Supplementary Fig. 2F, H ). These data suggested that deletion of METTL3 can suppress the EMT of cancer cells. To verify the role of m 6 A levels in EMT, we overexpressed ALKBH5, a key m 6 A demethylase of mammalian mRNA [37] , in HeLa cells. Our data showed that overexpression of ALKBH5 decreased mRNA of FN and MMP2 in HeLa cells (Supplementary Fig. 2G ). Western blot analysis showed that overexpression of ALKBH5 increased E-Cad while it decreased MMP2 and FN in HeLa cells (Fig. 1f ). Furthermore, TGF-β-induced downregulation of E-Cad and upregulation of FN were rescued in Mettl3 Mut/− HeLa (Fig. 1g ) and Mettl3 knockdown Huh7 (Supplementary Fig. 2H ) cells. The clinical roles of METTL3 were further investigated. TCGA data showed that expression of METTL3 in liver cancers was significantly higher than their matched adjacent normal tissues (Fig. 1h ). Moreover, the expression of METTL3 was negatively correlated with the CDH1 mRNA in 364 liver cancer patients (Fig. 1i ). It has been reported that TGF-β can induce the mRNA methylation in human embryonic stem cells (hESCs) via the interaction between Smad2/3 and the METTL3–METTL14–WTAP complex [38] . LC/MS/MS showed that the Smad2/3 inhibitor SB431542 (SB) can block TGF-β-induced upregulation of m 6 A in HeLa cells (Fig. 1j ). Together, our data indicated that the total m 6 A levels in mRNA may regulate EMT progression of cancer cells. Variations of m 6 A-regulated genes in cells undergoing EMT To investigate the variations of m 6 A modification in specific genes, we mapped m 6 A methylomes of HeLa cells undergoing EMT (EMT cells) by m 6 A sequencing (m 6 A-seq), with independent biological replicates. Principal component analysis (PCA) showed that two repeats of each sample clustered together, suggesting the good reproducibility among the two replicates of each group (Supplementary Fig. 3A ). GGAC motif was highly enriched within m 6 A sites in both control and EMT cells (Fig. 2a ). m 6 A peaks were especially abundant in the vicinity of start and stop codons (Fig. 2b ). Fig. 2 Variations of m 6 A-regulated genes in cells undergoing EMT. a Predominant consensus motif GGAC was detected in both the control and EMT cells in m 6 A-seq. b Density distribution of m 6 A peaks across mRNA transcripts. Regions of the 5′ untranslated region (5′UTR), coding region (CDS), and 3′ untranslated region (3′UTR) were split into 100 segments, then percentages of m 6 A peaks that fall within each segment were determined. c Proportion of m 6 A peak distribution in the 5′UTR, start codon, CDS, stop codon or 3′UTR region across the entire set of mRNA transcripts. d A cluster profiler identified the enriched gene ontology processes of 128 genes, which showed 1.5-fold m 6 A expression upregulation in EMT cells compared with control cells Full size image m 6 A-seq analysis identified 11,687 and 11,785 m 6 A peaks from 6836 to 7230 m 6 A-modified transcripts in control and EMT cells, respectively. In EMT cells, 4347 new m 6 A peaks and 4249 disappearing peaks were observed, while the remaining 7438 peaks were found in both control and EMT cells (Supplementary Fig. 3B ). For m 6 A-regulated genes, m 6 A-seq identified 569 new modifying genes and 472 genes loss of m 6 A modification in EMT cells, while the other 2357 genes were found in both control and EMT cells (Supplementary Fig. 3C ). The results indicated that EMT cells unique peaks and genes were expected to contain genuine targets. We further analyzed the total m 6 A distribution patterns of mRNAs according to the m 6 A-seq results. Similar patterns of the total m 6 A distribution in control and EMT cells were observed (Fig. 2c ), showing that m 6 A peaks were mainly enriched in exon regions. Furthermore, we investigated the distribution of unique EMT peaks. Compared with the 4249 missing peaks, which displayed identical distribution to total peaks, 4347 unique peaks in EMT cells showed a distinct pattern, in which a relative increase of m 6 A deposit appeared in both 5′ and 3′ UTR (Supplementary Fig. 3D ). Comparing the control to EMT cells, a total of 128 genes, showing a 1.5-fold m 6 A change in the expression level, were identified. Gene ontology (GO) enrichment analysis of these 128 genes indicated that a handful of genes were associated to the formation of the adherens junction and actin cytoskeleton in cancer cells undergoing EMT (Fig. 2d ). Collectively, the m 6 A-seq data revealed that m 6 A modifications occur on a handful of genes related to the cell junction, adhesion, and migration during EMT. 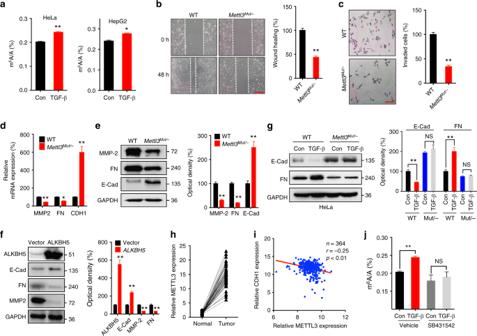Fig. 1 EMT in cancer cells is regulated by m6A levels of mRNAs.aHeLa and HepG2 cells were treated with or without 10 ng/ml TGF-β for 3 days, the m6A/A ratio of the total mRNA were determined by LC–MS/MS.bWound healing of wild-type (control) orMettl3Mut/−cells was recorded (left) and quantitatively analyzed (right).cWild-type orMettl3Mut/−cells were allowed to invade for 24 h and tested by CytoSelect™ 24-well Cell Invasion assay kits (8 µm, colorimetric format);d, emRNA (d) and protein (e) expressions of MMP2, FN, and E-Cad in wild-type andMettl3Mut/−HeLa cells were measured by qRT-PCR and western blot analysis, respectively.fHeLa cells were transfected with pcDNA/ALKBH5 or a vector control for 48 h, protein expression was determined by western blot analysis (left) and quantitatively analyzed (right).gWild-type orMettl3Mut/−cells were treated with or without 10 ng/ml TGF-β for 3 days, protein expression was determined by western blot analysis (left) and quantitatively analyzed (right).hThe expression of METTL3 in liver cancer and its matched adjacent normal tissues of 50 patients from TCGA database.iCorrelation between METTL3 and CDH1 in liver cancer patients (n= 364) from TCGA database.jHeLa cells were pretreated with or without Smad2/3 inhibitor SB431542 (10 μM) and then further treated with 10 ng/ml TGF-β for 3 days, the m6A/A ratio of the total mRNA were determined by LC–MS/MS. Data are presented as means ± SD from three independent experiments. *p< 0.05, **p< 0.01, NS, no significant, by Student’sttest. Red bar = 200 μm Snail is involved in m 6 A-regulated EMT in cancer cells To characterize potential targets involved in m 6 A-regulated EMT of cancer cells, we identified four genes overlapping between 84 EMT-related genes with key functions (listed in Supplementary Table 1 ) and the 61 m 6 A-regulated genes (greater than 2.0-fold m 6 A change) during EMT (Fig. 3a ). Among the four identified genes, Snail has been suggested as an important transcription factor controlling EMT [39] . Our data confirmed that SNAI1 mRNA was modified by m 6 A and showed significant enrichment of m 6 A in its CDS and 3′UTR regions during EMT progression (Fig. 3b, c ), which is consistent with the published reports using zebrafish embryonic cells [5] and human HEK293T cells [40] , [41] . By applying m 6 A RNA-immunoprecipitation (RIP) qPCR, we verified a 12-fold m 6 A antibody enriched SNAI1 mRNA (Fig. 3c ). During EMT, m 6 A levels of SNAI1 mRNA were significantly increased, and relative m 6 A enrichment fold in EMT cells was about 2.3-fold greater than in control cells (Fig. 3c ). However, neither m 6 A pull down enrichment nor m 6 A upregulation during EMT was observed for the negative candidate gene ZEB1 , which is another transcription factor of EMT as well (Supplementary Fig. 4A, B ). 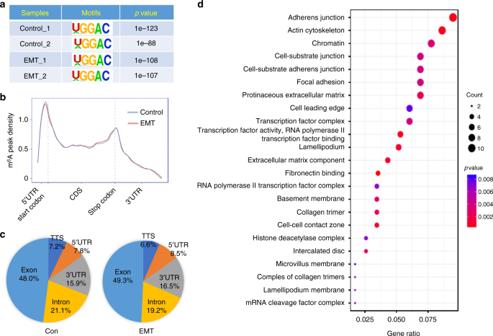Fig. 2 Variations of m6A-regulated genes in cells undergoing EMT.aPredominant consensus motif GGAC was detected in both the control and EMT cells in m6A-seq.bDensity distribution of m6A peaks across mRNA transcripts. Regions of the 5′ untranslated region (5′UTR), coding region (CDS), and 3′ untranslated region (3′UTR) were split into 100 segments, then percentages of m6A peaks that fall within each segment were determined.cProportion of m6A peak distribution in the 5′UTR, start codon, CDS, stop codon or 3′UTR region across the entire set of mRNA transcripts.dA cluster profiler identified the enriched gene ontology processes of 128 genes, which showed 1.5-fold m6A expression upregulation in EMT cells compared with control cells Fig. 3 Snail is involved in m 6 A-regulated EMT in cancer cells. a Overlapping of 2.0-fold m 6 A expression changes in EMT cells and EMT-related functional genes. 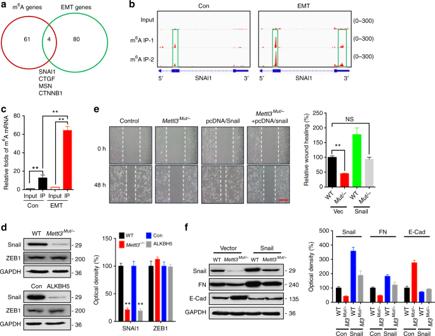Fig. 3 Snail is involved in m6A-regulated EMT in cancer cells.aOverlapping of 2.0-fold m6A expression changes in EMT cells and EMT-related functional genes.bm6A peaks were enriched in CDS and 3′UTRs of SNAI1 genes from m6A RIP-seq data. Squares marked increases of m6A peaks in cancer cells undergoing EMT;cm6A RIP-qPCR analysis of SNAI1 mRNA in the control and EMT undergoing HeLa cells.dProtein expression of Snail inMettl3Mut/−or AKLBH5 transfected (24 h) HeLa cells and the control.eThe wound healing of wild-type orMettl3Mut/−HeLa cells transfected with or without pcDNA/Snail for 48 h were recorded (left) and quantitatively analyzed (right).fWild-type orMettl3Mut/−HeLa cells were transfected with or without pcDNA/Snail for 48 h, expression of Snail, FN and E-Cad were measured by western blot analysis. Data are presented as means ± SD from three independent experiments. *p< 0.05, NS, no significant, by Student’sttest. Red bar = 200μm b m 6 A peaks were enriched in CDS and 3′UTRs of SNAI1 genes from m 6 A RIP-seq data. Squares marked increases of m 6 A peaks in cancer cells undergoing EMT; c m 6 A RIP-qPCR analysis of SNAI1 mRNA in the control and EMT undergoing HeLa cells. d Protein expression of Snail in Mettl3 Mut/− or AKLBH5 transfected (24 h) HeLa cells and the control. e The wound healing of wild-type or Mettl3 Mut/− HeLa cells transfected with or without pcDNA/Snail for 48 h were recorded (left) and quantitatively analyzed (right). f Wild-type or Mettl3 Mut/− HeLa cells were transfected with or without pcDNA/Snail for 48 h, expression of Snail, FN and E-Cad were measured by western blot analysis. Data are presented as means ± SD from three independent experiments. * p < 0.05, NS, no significant, by Student’s t test. Red bar = 200μm Full size image Next, we investigated protein expression of Snail in Mettl3 Mut/− and ALKBH5 overexpressing HeLa cells. We observed a decrease of Snail protein levels in HeLa (Fig. 3d ) and HepG2 (Supplementary Fig. 4C ) cells without changes in ZEB1 expression, in both contexts of deletion of METTL3 and overexpression of ALKBH5. To confirm the roles of m 6 A on Snail expression, we treated wild-type and Mettl3 Mut/− HeLa cells with TGF-β. 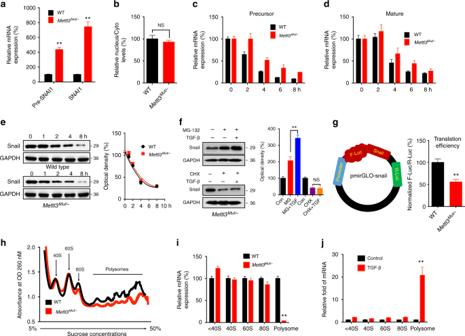Fig. 4 m6A triggers translation of Snail mRNA in cancer cells.aPrecursor and mature mRNA of SNAI1 in wild-type (WT) andMettl3Mut/−cells.bThe relative levels of the nuclear versus cytoplasmic SNAI1 mRNA in wild-type (WT) orMettl3Mut/−cells.c, dWild-type (WT) orMettl3Mut/−cells were pretreated with Act-D for 90 min, then precursor (c) or mature (d) SNAI1 mRNA were analyzed at indicated times.eWild-type (WT) orMettl3Mut/−cells were treated with CHX for the indicated times, and protein expression of Snail was analyzed by western blot analysis (left) and quantitatively analyzed (right);fMettl3Mut/−cells were pretreated with CHX or MG-132 for 6 h and then further treated with or without 10 ng/ml TGF-β for 48 h, the expression of Snail was detected by western blot analysis (left) and quantitatively analyzed (right).gWild-type (WT) orMettl3Mut/−cells were transfected with pmirGLO-Snail reporter for 24 h, and the translation efficiency of Snail is defined as the quotient of reporter protein production (F-luc/R-luc) divided by mRNA abundance7.hPolysome profiling of wild-type (WT) orMettl3Mut/−HeLa cells were analyzed.iAnalysis of Snail mRNA in non-ribosome portion (< 40S), 40S, 60S, 80S, and polysome for theMettl3Mut/−cells compared to control cells.jAnalysis of Snail mRNA in non-ribosome portion (< 40S), 40S, 60S, 80S, and polysome for EMT undergoing HeLa cells compared with control cells. Data are presented as means ± SD from three independent experiments. *p< 0.05, NS, no significant, by Student’sttest The results showed that TGF-β-induced expression of Snail was reduced in Mettl3 Mut/− cells (Supplementary Figure 4D ), which indicated that m 6 A participated in TGF-β-induced expression of Snail in cancer cells. Although the promotion roles of Snail in EMT and cancer progression have been well illustrated [27] , [42] , [43] , we further investigated the roles of Snail in m 6 A-triggered EMT of cancer cells. Overexpression of Snail attenuated the suppression of wound healing via METTL3 deletion in HeLa cells (Fig. 3e ). Consistently, overexpression of Snail antagonized the downregulation of FN and upregulation of E-Cad occurred in Mettl3 Mut/− cells (Fig. 3f ; Supplementary Fig. 4E ). These data suggested that Snail is involved in m 6 A-regulated EMT in cancer cells. m 6 A triggers translation of Snail mRNA in cancer cells The mechanisms regulating Snail expression through m 6 A methylation were further investigated. First, we tested the expression of precursor (pre-) and mature (mat-) mRNA of Snail. Surprisingly, expression of both precursor (pre-) and mature (mat-) mRNA of Snail in Mettl3 Mut/− cells were significantly enhanced (Fig. 4a ). However, there was no difference on promoter activity in wild-type and Mettl3 Mut/− cells (Supplementary Fig. 5A ), suggesting that transcription of Snail was not affected by m 6 A. By separating the nuclear and cytoplasmic RNAs (Supplementary Fig. 5B ), we found that there was no difference on subcellular localization of Snail mRNA between wild-type and Mettl3 Mut/− cells (Fig. 4b ). We treated wild-type and Mettl3 Mut/− HeLa cells with Act-D to block transcription. The results showed that half-life of both precursor (Fig. 4c ) and mature (Fig. 4d ) mRNA in wild-type cells were significantly shorter than in Mettl3 Mut/− cells. It indicated that m 6 A modification may trigger the splicing of precursor mRNA and the degradation of mature mRNA of Snail in cancer cells. This was confirmed by the results indicating that Snail was a target of YTHDF2 (Supplementary Fig. 5C ), which is responsible for m 6 A-mediated mRNA destabilization of transcripts [6] . Overexpression of YTHDF2 can decrease the expression and stability of mature Snail mRNA in HeLa cells (Supplementary Fig. 5D ). Fig. 4 m 6 A triggers translation of Snail mRNA in cancer cells. a Precursor and mature mRNA of SNAI1 in wild-type (WT) and Mettl3 Mut/− cells. b The relative levels of the nuclear versus cytoplasmic SNAI1 mRNA in wild-type (WT) or Mettl3 Mut/− cells. c, d Wild-type (WT) or Mettl3 Mut/− cells were pretreated with Act-D for 90 min, then precursor ( c ) or mature ( d ) SNAI1 mRNA were analyzed at indicated times. e Wild-type (WT) or Mettl3 Mut/− cells were treated with CHX for the indicated times, and protein expression of Snail was analyzed by western blot analysis (left) and quantitatively analyzed (right); f Mettl3 Mut/− cells were pretreated with CHX or MG-132 for 6 h and then further treated with or without 10 ng/ml TGF-β for 48 h, the expression of Snail was detected by western blot analysis (left) and quantitatively analyzed (right). g Wild-type (WT) or Mettl3 Mut/− cells were transfected with pmirGLO-Snail reporter for 24 h, and the translation efficiency of Snail is defined as the quotient of reporter protein production (F-luc/R-luc) divided by mRNA abundance [7] . h Polysome profiling of wild-type (WT) or Mettl3 Mut/− HeLa cells were analyzed. i Analysis of Snail mRNA in non-ribosome portion (< 40S), 40S, 60S, 80S, and polysome for the Mettl3 Mut/− cells compared to control cells. j Analysis of Snail mRNA in non-ribosome portion (< 40S), 40S, 60S, 80S, and polysome for EMT undergoing HeLa cells compared with control cells. Data are presented as means ± SD from three independent experiments. * p < 0.05, NS, no significant, by Student’s t test Full size image We observed increasing of mature SNAI1 mRNA levels while decreasing of protein levels of Snail in Mettl3 Mut/− cells, then we hypothesized that downregulation of Snail protein in Mettl3 Mut/− cells may be due to a difference on protein stability or translation efficiency. To verify this, both wild-type and Mettl3 Mut/− HeLa cells were treated with protein translation inhibitor cycloheximide (CHX). The results from western blot analysis showed that half-lives of Snail proteins were similar between wild-type and Mettl3 Mut/− HeLa cells (Fig. 4e ), suggesting that m 6 A-induced Snail expression was not related to protein stability. Furthermore, Mettl3 Mut/− HeLa cells were pretreated with MG132 to inhibit proteasome activity or CHX to block translation and then treated with TGF-β. The data showed that in the presence of CHX, but not MG-132, attenuated TGF-β-induced Snail expression in Mettl3 Mut/− HeLa cells (Fig. 4f ). We constructed the pmirGLO-Snail luciferase reporter by ligating Snail CDS to the mutiple cloning site (MCS) site. The dual-luciferase assay showed that translation efficiency of Snail in Mettl3 Mut/− HeLa cells was significantly lower than that in HeLa WT cells (Fig. 4g ). It indicated that m 6 A-induced Snail expression was related to regulation of translation. Next, we separated the RNA fractions: non-translating fraction (< 40 S), translation initiation fraction (including 40S ribosomes, 60S ribosomes, 80S monosomes, and < 80S) as well as translation active polysomes (> 80S) from wild-type and Mettl3 Mut/− HeLa cells by ribosome profiling (Fig. 4h ). Polysome profiling supported the decreases of 80S monosome assembly and polysomes in Mettl3 Mut/− cells (Fig. 4h ). qRT-PCR showed that Snail mRNA in translation-active polysomes (> 80S) of Mettl3 Mut/− cells were significantly lower than in wild-type cells (Fig. 4i ). In EMT cells, ribosome profiling was similar to that in wild-type cells (Supplementary Fig. 5E ). Remarkably, an increase of SNAI1 mRNA in polysomal fractions (> 80S) isolated from cancer cells undergoing EMT was observed (Fig. 4j ), indicating that translation of SNAI1 mRNA was improved during EMT process. To further confirm our observations, we targeted cap-independent/dependent translation initiation to investigate whether it was involved in m 6 A methylation-regulated SNAI1 translation. Both Mettl3 Mut/− and wild-type cells were treated with rapamycin, which inhibits cap-dependent but not cap-independent translation [44] . However, no obvious differences of Snail1 levels were observed between wild-type and Mettl3 Mut/− cells (Supplementary Fig. 5F ). Maintenance of Snail1 expression in the presence of rapamycin was not due to an increase of Snail1 protein stability, as co-treatment of wild-type cells with protein synthesis inhibitor CHX resulted in a rapid disappearance of Snail1 (Supplementary Fig. 5F ), suggesting that Snail expression was regulated through cap-independent translation [45] . m 6 A-methylated CDS regulates translation of Snail m 6 A-RIP-seq data showed that m 6 A peaks in CDS regions ranged from chr20:48,600,490 to 48,600,630, while in 3′UTR regions ranged from chr20: 48,604,770 to 48,605,060 (Fig. 3b ). One GGAC motif in CDS and two in 3′UTR of Snail mRNA were identified, as shown in Fig. 5a , which was consistent with positions and amounts of peaks identified by m 6 A RIP-seq. To characterize m 6 A methylation in Snail mRNA, we used m 6 A antibody to immunoprecipitated fragmented RNA isolated from HeLa cells (Supplementary Fig. 6A ). qRT-PCR showed that distributions of m 6 A methylation in Snail mRNA, from high to low, were: CDS, 3′UTR and 5′UTR, in wild-type HeLa cells (Supplementary Fig. 6B ). Consistently, the m 6 A enrichment of Snail CDS was significantly downregulated in Mettl3 Mut/− cells (Supplementary Fig. 6B ), suggesting that m 6 A methylation in CDS regions might be more dynamic than those in 3′UTR. To study the potential roles of m 6 A methylation on the SNAI1 3′UTR region, we generated luciferase reporters containing a firefly luciferase, followed by the wild-type SNAI1 3′UTR, mutant 1 or mutant 2 3′UTR (GG A C to GG C C, Fig. 5b ). The SNAI1 3′UTR-reporter luciferase assay showed that Snail 3′UTR from WT-3′UTR, mut1–3′UTR, and mut2–3′UTR had no translational difference between wild-type and Mettl3 Mut/− cells (Fig. 5c ). Consistently, co-transfection of ALKBH5 did not alter expression levels of WT-3′UTR, mut1–3′UTR, or mut2–3′UTR in HeLa cells (Supplementary Fig. 6C ). This suggested that m 6 A methylation on 3′UTR might not be involved in the m 6 A modification-regulated Snail expression. Fig. 5 m 6 A methylated CDS regulates translation of Snail. a Schematic representation of positions of m 6 A motifs within Snail mRNA. b Schematic representation of mutated (GG A C to GG C C) 3’UTR of pmirGLO vector to investigate the m 6 A roles on Snail expression. c pmirGLO-3′UTR or pmirGLO-3′UTR-Mut1/2 reporter was transfected into wild-type or Mettl3 Mut/− HeLa cells for 24 h. d pcDNA-Snail-CDS-WT, pcDNA-Snail-mut1/2, or pcDNA/ZEB1 were transfected into HeLa cells for 24 h. Protein expression was measured by western blot analysis (left) and quantitatively analyzed (right). e Schematic representation of mutation in CDS to investigate the m 6 A roles on Snail expression. f After transfected with pcDNA-Snail-CDS-WT or pcDNA-Snail-mut1/2, HeLa cells were further treated with or without 10 ng/ml TGF-β for 48 h. The expression of Snail was measured by western blot analysis (left) and quantitatively analyzed (right). g YTHDF1 RIP-qPCR analysis of SNAI1 mRNA in wild-type or Mettl3 Mut/− HeLa cells. h Binding of YTHDF1 with the CDS or 3’UTR in wild-type or Mettl3 Mut/− cells were analyzed by YTHDF1 RIP-qPCR using fragmented RNA. i After pre-transfected with siNC or si-YTHDF1 for 12 h, HeLa cells were further treated with or without 10 ng/ml TGF-β for 48 h. Protein expression was measured by western blot analysis (left) and quantitatively analyzed ( right ). j eEF-1 and eEF-2 RIP-qPCR analysis of SNAI1 mRNA in wild-type or Mettl3 Mut/− HeLa cells. k Binding between YTHDF1 with eEF-1 or eEF-2 in wild-type or Mettl3 Mut/− HeLa cells was checked by immunoprecipitation (left) and quantitatively analyzed (right). Data are presented as means ± SD from three independent experiments. * p < 0.05, NS, no significant, by Student’s t test Full size image We then investigated whether m 6 A methylation in CDS can regulate the expression of Snail. First, we generated an expression construct containing Snail CDS alone. We co-transfected Snail CDS with pcDNA/ZEB1, expression of which was not regulated by m 6 A methylation, to normalize the transfection efficiency. The results showed that expression of Snail in Mettl3 Mut/− cells remarkably decreased, while expression of ZEB1 was not affected, indicating that m 6 A methylation in CDS was critically involved in m 6 A-mediated Snail expression (Fig. 5d ). Second, we mutated the potential m 6 A motif GG A C to GG C C (CDS-mut1). Accordingly, the nearby GG A A was mutated to GG C A for comparison (CDS-mut2, both mutants were located at chr20: 48,600,490–48,600,630, Fig. 5e ). Our data showed that Snail level was partially recruited in Mettl3 Mut/− cells overexpressing pcDNA-Snail-CDS-mut1, but not CDS-mut2 (Fig. 5d ). HeLa cells transfected with pcDNA-Snail-CDS-WT or pcDNA-Snail-CDS-mut1/mut2 were further treated with TGF-β. Western blot results showed that TGF-β-induced Snail expression of pcDNA-Snail-CDS-mut1 was lower than pcDNA-Snail-CDS-WT or pcDNA-Snail-CDS-mut2 (Fig. 5f ). Together, our data indicated that m 6 A in SNAI1 CDS was the main location for expression regulation. YTHDF1, acting as a m 6 A “reader”, recognizes m 6 A methylated mRNA and promotes the translation of its targets [7] . In order to verify whether YTHDF1 participates in m 6 A methylation of SNAI1 mRNA, RIP-qPCR was used to investigate the interaction between SNAI1 mRNA and YTHDF1. Our data showed that YTHDF1 enriched in SNAI1 mRNA remarkably, while this relative enrichment (IP vs. input) was significantly suppressed in Mettl3 Mut/− cells (Fig. 5g ). The results of RIP-PCR further revealed that YTHDF1 preferred to interact with the CDS region of Snail mRNA rather than 3′UTR region (Fig. 5h ). In Mettl3 Mut/− cells, binding between YTHDF1 with CDS, but not 3′UTR, of SNAI1 mRNA, was significantly decreased in comparison with HeLa cells. To confirm the roles of YTHDF1 in m 6 A-regulated Snail expression, we knocked down expression of YTHDF1 in HeLa cells (Supplementary Fig. 6D ). Our data showed that si-YTHDF1 attenuated TGF-β-induced expression of Snail in HeLa cells (Fig. 5i ). Similarly, overexpression of YTHDF1 increased protein expression of Snail in both HeLa and HepG2 cells, while it had no effect on the expression of ZEB1 (Supplementary Fig. 6E ). Since the translation elongation in eukaryotes is carried out with two elongation factors: eEF-1 and eEF-2 [46] , we measured the variation of eEF-1- and eEF-2-binding Snail mRNA in Mettl3 Mut/− HeLa cells. Our data showed that the binding between Snail mRNA and eEF-2, but not eEF-1, in Mettl3 Mut/− HeLa cells was significantly less than that in HeLa cells (Fig. 5j ). Furthermore, co-IP analysis indicated that the binding between YTHDF1 and eEF-2, while not eEF-1, was significantly decreased in Mettl3 Mut/− HeLa cells compared with that in WT HeLa cells (Fig. 5k ). This data suggested that YTHDF1 and eEF-2 are likely responsible for the m6A-induced translation elongation of Snail mRNA in cancer cells. m 6 A regulates in vivo cancer progression We used three animal cohorts to study the potential effects of m 6 A methylation on cancer cells in vivo metastasis. First, both sh-control and sh-Mettl3 Huh7 cells were injected subcutaneously into nude female mice. Mice were killed when the tumor volumes were about 100 mm 3 for each group. IHC results showed that METTL3 depletion led to a lower level of Snail, FN, and Vim in xenograft tumor tissues (Fig. 6a ), which suggested that the knockdown of METTL3 can decrease the EMT potential and Snail expression of Huh7 cells when the tumor volumes were comparable. To further determine the impacts of m 6 A methylation on in vivo metastasis, both sh-control and sh-Mettl3 Huh7 cells were injected into the BALB/c nude mice, respectively, by tail vein injection to analyze lung colonization. Eight weeks after injection, the experiment was terminated and lungs were analyzed to report the presence of metastatic tumors. As shown in Fig. 6b , the number of lung tumors derived from METTL3 knockdown Huh7 cells was significantly decreased compared with control cells, suggesting that METTL3 deficiency suppressed tumor metastasis in vivo. To investigate whether Snail was involved in m 6 A regulated in vivo metastasis, HeLa WT, Mettl3 Mut/− HeLa, HeLa Snail , and Mettl3 Mut/− HeLa Snail stable cells were injected into nude mice via intravenous tail vein. In vivo data showed that the number of lung tumors derived from Mettl3 Mut/− HeLa cells was significantly decreased compared with HeLa WT cells; however, overexpression of Snail can attenuate the suppression effect of Mettl3 Mut/− HeLa cells on in vivo lung colonization (Fig. 6c ). It suggested that Snail was involved in the in vivo metastasis effect of METTL3. Fig. 6 m 6 A methylation regulates in vivo cancer progression. a IHC (Snail, FN, and Vim)-stained paraffin-embedded sections obtained from sh-control and sh-Mettl3 Huh7 xenografts when the tumor volumes were about 100 mm 3 for each group. b The sh-control and sh-Mettl3 Huh7 cells were injected into the nude mice by tail vein injection. Representative images of metastatic lung tumors and the H&E staining results were shown (left), and the number of lung tumors was quantitatively analyzed (right). c HeLa WT, Mettl3 Mut/− HeLa, HeLa Snail , and Mettl3 Mut/− HeLa Snail stable cells were injected into the nude mice by tail vein injection. Representative images of metastatic lung tumors and the H&E staining results were shown (left), and the number of lung tumors was quantitatively analyzed (right). d Expression of YTHDF1 in paired human liver ( n = 26) cancer tissues and adjacent normal mucosa tissues from TCGA database. e YTHDF1 expression in liver cancers of T1 ( n = 153), T2 ( n = 77), T3 ( n = 65), and T4 ( n = 13) stages from TCGA database. f Correlation between YTHDF1 and SNAI1 in liver cancer patients ( n = 80) from TCGA database. g METTL3 expression in HCC tumor tissues ( n = 35), liver cirrhosis tissues ( n = 13), and normal liver tissues ( n = 10) from Oncomine database (Wurmbach liver cancers). h Correlation between Mettl3 and Snail protein in liver cancer patients (100) by use of tissue microarray (CS03–01–008, Alenabio, Xian, Shanxi, China). i , j , k Kaplan–Meier survival curves of OS based on METTL3 ( i ), YTHDF1 ( j ), or SNAI1 ( k ) mRNA expression in HCC patients. The log-rank test was used to compare differences between two groups. Data are presented as means ± SD from three independent experiments. * p < 0.05, ** p < 0.01, NS, no significant, by one-way ANOVA with Bonferroni test. Red bar = 200 μm Full size image Our data suggested that knockdown of METTL3 can decrease the expression of Snail and the in vitro invasion and EMT of HepG2 and Huh7 cells (Supplementary Figs. 2E, 2F , 4C ), we then questioned the possibility of a link between m 6 A methylation and clinical development of liver cancer. Increased expression of METTL3 (Fig. 1h ) and YTHDF1 (Fig. 6d ) was observed in liver cancer tissues as compared with matched adjacent normal tissues. Significant rising expression levels of YTHDF1 from T1 to T4 stage of liver cancer tissues were observed (Fig. 6e ), implying an increasing tendency of YTHDF1 expression during malignant transformation. In addition, expression of YTHDF1 was positively correlated with the SNAI1 mRNA in liver (Fig. 6f ) cancer patients. Rising expression levels of METTL3 from the normal liver to cirrhosis to liver cancer tissues were observed (Fig. 6g ). Considering that Mettl3 induced Snail via translation, we checked their protein expression in 100 cases of liver cancer tissues by use of tissue microarray. IHC analysis confirmed that the expression of Mettl3 was significantly ( p < 0.05, t test) positively associated with that of Snail in the measured 100 liver cancers (Fig. 6h ). Using the online bioinformatics tool Kaplan–Meier plotter [47] , we found that liver cancer patients with increased expression of METTL3 (Fig. 6i ), YTHDF1 (Fig. 6j ), and Snail (Fig. 6k ) showed reduced overall survival (OS). Increasing evidences suggested that m 6 A mRNA modification participates in a number of biological functions and in progression of cancer cells [15] , [20] , [21] . In this study, we demonstrated that m 6 A can regulate the progression of EMT and expression of Snail. In brief, m 6 A levels in mRNA of cancer cells undergoing EMT increased significantly compared with control cells. Deletion of METTL3 or overexpression of ALKBH5 suppressed the in vitro migration, invasion, and EMT of cancer cells. m 6 A-seq and GO analysis showed that genes related to cell migration and adherens junctions are dynamically regulated by m 6 A during EMT. Particularly, Snail, a key transcription factor of EMT, was m 6 A methylated in its CDS and 3′UTR regions. Gain and loss of function studies revealed that m 6 A in CDS of Snail can trigger its translation elongation via interaction with YTHDF1 and eEF-2. Deletion of METTL3 suppressed the in vivo metastasis of cancer cells, which could be attenuated by the overexpression of Snail. Consistently, clinical data showed that tumor tissues contained higher METTL3 and YTHDF1 levels than adjacent normal tissues, which induced worse prognosis for liver cancer patients. The roles of mRNA modification in controlling the cancer progression have just begun to be studied. FTO, the first characterized m 6 A demethylase, has been reported to enhance leukemic oncogene-mediated cell transformation and leukemogenesis via regulation of expression of its targets, such as ASB2 and RARA , by reducing their m 6 A levels [20] . Another m 6 A demethylase ALKBH5 can also trigger tumorigenicity of glioma stem-like cells (GSC) by sustaining FOXM1 expression and cell proliferation [23] . METTL3, which is the methyltransferase of mRNA m 6 A, exhibits several functions in cancer cells, such as: maintaining myeloid leukemia [48] , promoting liver cancer progression [49] , playing essential role in GSC maintenance and radioresistance [50] , positively regulating proliferation of hematopoietic stem/progenitor cells (HSPCs) [51] , and triggering the translation in cancer cells [52] . Contradictorily, METTL3 acts as a tumor suppressor in renal cell carcinoma [53] . METTL14, which forms a stable heterodimer core complex with METTL3 to function in cellular m 6 A deposition, can suppress metastatic potential by modulating the primary microRNA 126 processing in an m 6 A-dependent manner [54] . In this study, we provided the causative link between mRNA m 6 A methylation and EMT. We found that levels of m 6 A in mRNA increased in cancer cells undergoing EMT, while targeted deletion of METTL3 impaired the migration and EMT of cancer cells. GO analysis revealed that modulation of mRNA m 6 A levels impacted multiple aspects of cancer progression, including migration, self-renewal, and tumorigenesis. Our results described the roles of m 6 A and METTL3 in cancer progression, and also created the possibility to develop therapeutic strategies against cancer metastasis by targeting m 6 A modification and its related targets. m 6 A modification modulates all stages in the life cycle of RNA, such as RNA processing, nuclear export, and translation modulation [13] , [55] . First, splicing regulators and a m 6 A “reader” HNRNPC could affect the abundance as well as alternative splicing of target mRNAs in a m 6 A switch-regulated manner [56] . Second, m 6 A was found to promote RNA export from the nucleus to cytoplasm, which was evidenced by the fact that METTL3 knockdown delayed mRNA export [57] , while inhibition of ALKBH5 enhanced mRNA export to the cytoplasm [37] . Third, m 6 A modification can trigger mRNA degradation by promoting deadenylation of RNAs through the first characterized m 6 A “reader” protein YTHDF2 [6] . Half-life of Snail mRNA in Mettl3 Mut/− cells was significantly longer than in control cells, which indicated a negative impact of m 6 A on mRNA stability. FTO mediated repression of ASB2 and RARA stability [20] and ALKBH5 modulated FOXM1 expression via m 6 A modifications in 3′UTR of targets [23] . However, our luciferase/mutation assays showed that m 6 A in 3′UTR had no effect on Snail protein expression, suggesting that m 6 A regulation on mRNA stability is more complicated than expected and could be related to target or location specificity. We revealed that m 6 A triggered translation of Snail mRNA through YTHDF1 and eEF-2 binding with methylated mRNA. YTHDF1 interacts with EIF3 to promote the rate-limiting step of translation for m 6 A-modified mRNAs by increasing their association with polysomes [7] . Our data showed that YTHDF1 prefers to bind with the CDS of Snail mRNA and then triggers its association with polysome in cancer cells undergoing EMT. The mutation of GGAC motif can partially rescue m 6 A-regulated translation. Similarly, in METTL3 deletion acute myeloid leukemia (AML) cells, c-MYC, BCL2, and PTEN protein expression were reduced despite a 2–5 log 2 -fold increase in mRNA expression [51] . A specific shift of SP1 and SP2 transcripts toward lower-molecular-weight polysomes has been observed in METTL3 depletion cancer cells [48] . Alternatively, METTL3 can localize to polysomes and functionally associate with translation initiation factors to promote translation in an YTHDF1-independent manner [52] . In Mettl3 Mut/− cells, the binding between Snail mRNA and eEF-2 or between YTHDF1 and eEF-2 was decreased. eEF-2 is essential for the GTP-dependent translocation of the ribosome along mRNA [58] . Our results also showed that m 6 A-regulated Snail translation is cap-independent, which was evidenced by the fact that rapamycin had no effect on Snail expression in wild-type and Mettl3 Mut/− cells. However, to determinate if promoter-bound METTL3 augments translation [48] will need further studies. In summary, we provide compelling in vitro and in vivo evidences demonstrating that m 6 A can regulate the progression of EMT, cancer metastasis, and Snail translation. Our present research provided the mechanism of regulation of cancer progression by modulation of EMT through RNA m 6 A modification. It should be noted that the effects of Mettl3-modified Snail mRNA might be heterogeneous in different tumor models, further, Snail is not always associated with the induction of mesenchymal features [59] , [60] and EMT is not necessary for the generation of metastases in some cancers [59] , [61] . The roles of m 6 A in cancer metastasis and Snail expression in other types of cancer need further investigation. Cell culture, treatments, and transfection Human cancer HeLa, HepG2, Huh7, and A549 cells were purchased from the American Type Culture Collection (ATCC, Manassas, VA, USA) and maintained in our lab with Dulbecco’s modified Eagle medium (DMEM, GIBCO, Carlsbad, CA, USA) with 10% fetal bovine serum (FBS) and 1% penicillin/streptomycin (Invitrogen). Cells were routinely tested for mycoplasma contamination using MycoAlert Mycoplasma Detection Kit. To establish the model of cancer cells undergoing EMT, cells were treated with 10 ng/ml TGF-β for 3 days. To generate Mettl3 Mut/− HeLa cells, the CRISPR-cas9 editing system was used according to the published protocol [36] . The sh-Control and sh-Mettl3 Huh7 cells were kindly provided by Prof Jun Cui at Sun Yat-sen University. To generate Snail stable overexpression cells, the wild-type and Mettl3 Mut/− HeLa cells were transfected with pcDNA/Snail or vector control and via liposome-mediated transfection. The transfected cells were selected with G418 (700 μg/ml) for 2 weeks. The survived cells were picked out and seeded into 96-well plate for formation of cell clones and further expansion. The expanded monoclonal cell populations were named as HeLa WT, Mettl3 Mut/− HeLa, HeLa Snail , and Mettl3 Mut/− HeLa Snail cells, respectively. The expression of Snail and Mettl3 was checked by western blot analysis. For overexpression of METTL3, Snail, ALKBH5, YTHDF1, or YTHDF2, cells were transfected with plasmids by lipofectamine 2000 according to the manufacturers’ instructions. For YTHDF1 or METTL3 knockdown, three synthesized duplex RNAi oligos targeting human YTHDF1 or METTL3 mRNA sequences from Sigma were used. The most efficient one was selected for following studies. A scrambled duplex RNA oligo (5′-UUCUCCGAACGUGUCACGU) was used as a RNA negative control (si-NC). Lipofectamine RNAiMAX (Invitrogen) was used for siRNA transfection. Working concentration for siRNA was 50 nM. Wound-healing and in vitro invasion assay For wound-healing assay, cells were seeded and cultured until a 90% confluent monolayer was formed. Cells were then scratched by a sterile pipette tip and treated as indicated in the text in the FBS-free medium. Cell migration distances into the scratched area were measured in 10 randomly chosen fields under a microscope. Transwell assay was conducted using CytoSelect™ 24-well Cell Invasion assay kits. Briefly, polycarbonate filters (8-μm pore size, Corning) coated with 50% Matrigel (BD bioscience, Bedford, MA) were used to separate upper and lower chambers. In total, 1 × 10 5 cells in 200 μl of the culture medium (supplemented with 0.1% FBS) were added into the upper chamber, while 600 μl medium supplemented with 10% FBS were added into the lower chamber and served as a chemotactic agent. After incubation, cells invading into the lower chamber were fixed, stained, and counted under the upright microscope (five fields per chamber). RNA extraction and real-time PCR for gene expression RNA extraction with Trizol (Invitrogen) and real-time PCR were performed according to the protocol used in our previous study [18] . Primers of targeted genes were as follow: GAPDH, forward 5′-GTC TCC TCT GAC TTC AAC AGC G-3′ and reverse 5′-ACC ACC CTG TTG CTG TAG CCA A-3′ MMP2, forward 5′-AGC GAG TGG ATG CCG CCT TTA A-3′ and reverse 5′-CAT TCC AGG CAT CTG CGA TGA G-3′ FN1, forward 5′-ACA ACA CCG AGG TGA CTG AGA C-3′ and reverse 5′-GGA CAC AAC GAT GCT TCC TGA G-3′ CDH1, forward 5′-GCC TCC TGA AAA GAG AGT GGA AG-3′ and reverse 5′-TGG CAG TGT CTC TCC AAA TCC G-3′ Pre-Snail, forward 5′-GGG ACA GTT GAA CCC CTC AG-3′ and reverse 5′-GGA GTC AAT GAG GAC CGC AA-3′ (mat-) Snail, forward 5′-TGC CCT CAA GAT GCA CAT CCG A-3′ and reverse 5′-GGG ACA GGA GAA GGG CTT CTC-3′ ZEB1, forward 5′-GGC ATA CAC CTA CTC AAC TAC GG-3′ and reverse 5′-TGG GCG GTG TAG AAT CAG AGT C-3′ METTL3, forward 5′-CTA TCT CCT GGC ACT CGC AAG A-3′ and reverse 5′-GCT TGA ACC GTG CAA CCA CAT C-3’YTHDF1, forward 5′- CAA GCA CAC AAC CTC CAT CTT CG-3′ and reverse 5′-GTA AGA AAC TGG TTC GCC CTC AT-3′. For quantitative RT-PCR, GAPDH was used as endogenous control for the cytoplasmic RNA, while 18S RNA was selected as endogenous control for the nuclear RNA. Western blot analysis Western blot analysis was performed as previously described [32] . The antibodies used in this study were MMP2 (Bioworld, BS1236, 1:500), FN (Novus, NBP1-91258, 1:500), E-Cad (Bioworld, 3195S, 1:500), ALKBH5 (Abcam, ab69325, 1:500), Snail (Bioworld, BS1853, 1:500), ZEB1 (Millipore, ABD53, 1:1000), eEF-1 (Proteintech, 11402–1-AP, 1:500), eEF-2 (Proteintech, 20107–1-AP, 1:500), YTHDF1 (Abcam, ab99080, 1:500), and GAPDH (BOSTER, BM3876, 1:1000). The uncropped gel images are shown in Supplementary Figs 7 and 8 . LC–MS/MS assay mRNA was purified from the total RNA using oligo dT magnetic beads. About 200 ng of purified mRNAs were incubated with nuclease P1 (0.5 U, Sigma) in 25 -μl reaction system containing 10 mM NH 4 OAc (pH = 5.3) at 42 °C for 1 h, followed by addition of NH 4 HCO 3 (1 M, 3 μL) and alkaline phosphatase (1 μL, 1 U/μL; Sigma) and incubation at 37 °C for 2 h. After neutralized by 1 μl HCl (3 M), samples were diluted to 50 μl and filtered by 0.22 μm filter (Millipore). All samples (10 μl for each injection) were separated by a C18 column (Agilent) using reverse-phase ultra-performance liquid chromatography and analyzed by an Agilent 6410 QQQ triple-quadrupole LC mass spectrometer using a positive electrospray ionization mode. All nucleosides were quantified by use of retention time and ion mass transitions of 268.0 to 136.0 (A) and 282.1 to 150.0 (m 6 A). Quantification was calculated using standard curves from standards running in the same batch. Ratio of m 6 A to A was calculated based on calibration curves. Dot-blot assay mRNA was enriched using GenElute messenger RNA (mRNA) Miniprep Kit (Sigma‐Aldrich) and RiboMinus Transcriptome Isolation Kit (human/mouse; ThermoFisher Scientific). After 5 min of denaturation at 70 °C, equal amounts of serial-diluted mRNA were added into an Amersham Hybond N + membrane (GE Healthcare) and cross-linked into auto-cross-linker three times under auto-cross-linking mode. Membrane was blocked with 5% milk in 1× PBST for 1 h at room temperature and then was inducted with anti‐m 6 A antibody (SySy) overnight (4 °C). Membrane was washed according to the standard protocol. Horseradish peroxidase-conjugated anti-rabbit immunoglobulin G (Cell Signaling Technology) was diluted 1:5000 and incubated with the membranes for 1 h at room temperature. Membranes were developed with a 3,3′‐diaminobenzidine peroxidase substrate kit (Yeasen Biotechnology, Shanghai, China) to detect the signal. m 6 A sequencing (m 6 A-seq) and data analysis The total polyadenylated RNA was isolated from HeLa cells treated with or without 10 ng/ml TGF-β for 3 days using TRIZOL reagent followed by isolation through FastTrack MAGMaxi mRNA isolation kit (Invitrogen). RNA fragmentation, m 6 A-seq, and library preparation were performed according to the manufacturer’s instructions and previously published protocol [7] . NEBNext Ultra Directional RNA Library Prep Kit (New England BioLabs, Ipswich, MA, USA) was used for library preparation. Each experiment was conducted with two biological replicates. m 6 A-seq data were analyzed according to protocols described before [7] . Significant peaks with FDR < 0.05 were annotated to RefSeq database (hg19). Sequence motifs were identified by using Homer. Gene expression was calculated by Cufflinks using sequencing reads from input samples. Cuffdiff was used to find DE genes. m 6 A-RT-PCR m 6 A-RT-PCR was conducted according to previously described protocol with a slight modification [20] . Briefly, the total RNA was extracted using Trizol and fragmented by RNA fragmentation reagents (Thermo, AM8740) or not. After saving 50 ng of the total RNA as input, the remaining RNAs (2 μg) were used for m 6 A-immunoprecipitation with m 6 A antibody (Synaptic Systems) in 500 μL of IP buffer (150 mM NaCl, 0.1% NP-40, 10 mM Tris, pH 7.4, 100 U RNase inhibitor) to obtain m 6 A pull down portion (m 6 A IP portion). m 6 A RNAs were immunoprecipitated with Dynabeads ® Protein A (ThermoFisher Scientific) and eluted twice with elution buffer (5 mM Tris-HCL pH 7.5, 1 mM EDTA pH 8.0, 0.05% SDS, 20 mg/ml Proteinase K). m 6 A IP RNAs were recovered by ethanol precipitation, and RNA concentration was measured with Qubit ® RNA HS Assay Kit (ThermoFisher Scientific). Then 2 ng of the total RNA and m 6 A IP RNA were used as templates in qRT-PCR, as described above. RT-PCR for Snail was conducted using the following primers: 5′UTR, forward 5′-CGG CCT AGC GAG TGG TTC T-3′ and reverse 5′-TCG AGG CAC TGG GGT CG-3′ CDS, forward 5′-GCC AAT TGC CTG GGC CTC C-3′ and reverse 5′-GGC TGG GAG CCT TTC CCA CTG-3′ 3′UTR, forward 5′-TGG ATA CAG CTG CTT TGA GC-3′ and reverse 5′-TGT GAG GGG AGT GGG GTC-3′. Housekeeping gene HPRT1 was chosen as internal control since HPRT1 mRNA did not have m 6 A peaks from m 6 A profiling data [6] . RIP–RT-PCR For RNA immunoprecipitation, cells were irradiated twice with 400 mJ/cm 2 at 254 nm by Stratalinker on ice and lysed in high salt lysis buffer (300 mM NaCl, 0.2% NP-40, 20 mM Tris-HCl PH 7.6, 0.5 mM DTT, protease inhibitor cocktail (1 tablet/50 ml), and RNase inhibitor (1:200)) at 4 °C for 30 min. After treatment with, or without, 1 U RNase T1 for 15 min at 24 °C, 10% supernatant was collected as input. 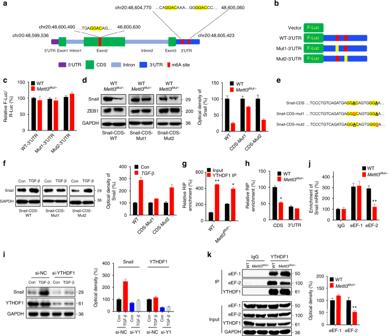Fig. 5 m6A methylated CDS regulates translation of Snail.aSchematic representation of positions of m6A motifs within Snail mRNA.bSchematic representation of mutated (GGAC to GGCC) 3’UTR of pmirGLO vector to investigate the m6A roles on Snail expression.cpmirGLO-3′UTR or pmirGLO-3′UTR-Mut1/2 reporter was transfected into wild-type orMettl3Mut/−HeLa cells for 24 h.dpcDNA-Snail-CDS-WT, pcDNA-Snail-mut1/2, or pcDNA/ZEB1 were transfected into HeLa cells for 24 h. Protein expression was measured by western blot analysis (left) and quantitatively analyzed (right).eSchematic representation of mutation in CDS to investigate the m6A roles on Snail expression.fAfter transfected with pcDNA-Snail-CDS-WT or pcDNA-Snail-mut1/2, HeLa cells were further treated with or without 10 ng/ml TGF-β for 48 h. The expression of Snail was measured by western blot analysis (left) and quantitatively analyzed (right).gYTHDF1 RIP-qPCR analysis of SNAI1 mRNA in wild-type orMettl3Mut/−HeLa cells.hBinding of YTHDF1 with the CDS or 3’UTR in wild-type orMettl3Mut/−cells were analyzed by YTHDF1 RIP-qPCR using fragmented RNA.iAfter pre-transfected with siNC or si-YTHDF1 for 12 h, HeLa cells were further treated with or without 10 ng/ml TGF-β for 48 h. Protein expression was measured by western blot analysis (left) and quantitatively analyzed (right).jeEF-1 and eEF-2 RIP-qPCR analysis of SNAI1 mRNA in wild-type orMettl3Mut/−HeLa cells.kBinding between YTHDF1 with eEF-1 or eEF-2 in wild-type orMettl3Mut/−HeLa cells was checked by immunoprecipitation (left) and quantitatively analyzed (right). Data are presented as means ± SD from three independent experiments. *p< 0.05, NS, no significant, by Student’sttest 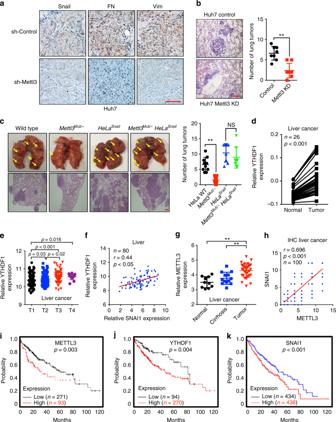Fig. 6 m6A methylation regulates in vivo cancer progression.aIHC (Snail, FN, and Vim)-stained paraffin-embedded sections obtained from sh-control and sh-Mettl3 Huh7 xenografts when the tumor volumes were about 100 mm3for each group.bThe sh-control and sh-Mettl3 Huh7 cells were injected into the nude mice by tail vein injection. Representative images of metastatic lung tumors and the H&E staining results were shown (left), and the number of lung tumors was quantitatively analyzed (right).cHeLa WT,Mettl3Mut/−HeLa, HeLaSnail, andMettl3Mut/−HeLaSnailstable cells were injected into the nude mice by tail vein injection. Representative images of metastatic lung tumors and the H&E staining results were shown (left), and the number of lung tumors was quantitatively analyzed (right).dExpression of YTHDF1 in paired human liver (n= 26) cancer tissues and adjacent normal mucosa tissues from TCGA database.eYTHDF1 expression in liver cancers of T1 (n= 153), T2 (n= 77), T3 (n= 65), and T4 (n= 13) stages from TCGA database.fCorrelation between YTHDF1 and SNAI1 in liver cancer patients (n= 80) from TCGA database.gMETTL3 expression in HCC tumor tissues (n= 35), liver cirrhosis tissues (n= 13), and normal liver tissues (n= 10) from Oncomine database (Wurmbach liver cancers).hCorrelation between Mettl3 and Snail protein in liver cancer patients (100) by use of tissue microarray (CS03–01–008, Alenabio, Xian, Shanxi, China).i,j,kKaplan–Meier survival curves of OS based on METTL3 (i), YTHDF1 (j), or SNAI1 (k) mRNA expression in HCC patients. The log-rank test was used to compare differences between two groups. Data are presented as means ± SD from three independent experiments. *p< 0.05, **p< 0.01, NS, no significant, by one-way ANOVA with Bonferroni test. Red bar = 200 μm Remaining supernatant was incubated with anti-YTHDF1 antibody, or IgG-conjugated protein A/G Magnetic Beads in 500 mL 1× IP buffer supplemented with RNase inhibitors at 4 °C overnight. Bound RNAs were immunoprecipitated with beads and treated with 100 µl of elution buffer (5 mM Tris-HCL pH 7.5, 1 mM EDTA pH 8.0, 0.05% SDS, 20 mg/ml Proteinase K) for 2 h at 50 °C, and RNA was recovered with phenol:chloroform extraction followed by ethanol precipitation. IP enrichment ratio of a transcript was calculated as ratio of its amount in IP to that in the input, yielded from same amounts of cells. RNA stability To measure RNA stability in HeLa wild-type and Mettl3 Mut/− cells, actinomycin D (Act-D, Catalog #A9415, Sigma, USA) at 5 μg/ml was added to cells. After incubation at the indicated times, cells were collected, and RNA was isolated for real-time PCR. Half-life (t1/2) of precursor and mature Snail mRNA were calculated using ln2/slope and GAPDH was used for normalization. Protein stability To measure protein stability, HeLa wild-type and Mettl3 Mut/− cells were treated with cycloheximide (CHX, final concentration 100 μg/ml) during indicated times. The expression of Snail was measured through western blot analysis. Snail promoter activity assay Promoter activity of Snail in HeLa wild-type and Mettl3 Mut/− cells was measured according to our previously described protocol [62] . Briefly, cells were transfected with pGL3-Basic-Snail-luc containing sequence −797/ + 59 of Snail promoter. Transfection efficiency was normalized by co-transfection with pRL-TK. Transcriptional activity was determined by a luminometer, using a dual-luciferase assay kit. The results were displayed as the ratios between the activity of reporter plasmid and pRL-TK. Luciferase reporter assay Luciferase assay was performed using reporter lysis buffer (Catalog #E3971, Promega, USA) and luciferase assay reagent according to the manufacturer’s instructions. Briefly, HeLa wild-type and Mettl3 Mut/− cells were transfected with pmiRGLO, pmiRGLO-WT-3′UTR, pmiRGLO-Mut1-3′UTR, or pmiRGLO-Mut2-3′UTR in a 12-well plate. After transfection for 6 h, each cell line was re-seeded into a 96-well plate. After 24 h incubation, cells were analyzed with the Dual-Glo Luciferase Assay system (Promega). Renilla Luciferase (R-luc) was used to normalize firefly luciferase (F-luc) activity to evaluate reporter translation efficiency. Experimental animals and xenograft models Female BALB/c nude mice (4-week-old) were purchased from Sun Yat-sen University (Guangzhou, China) Animal Center and raised under pathogen-free conditions. All animal experiments complied with Zhongshan School of Medicine Policy on Care and Use of Laboratory Animals. For subcutaneous transplanted model, sh-control and sh-METTL3 Huh7 cells (5 × 10 6 per mouse, n = 5 for each group) were diluted in 200 μL of PBS + 200 μL Matrigel (BD Biosciences) and subcutaneously injected into immunodeficient female mice to investigate tumor growth. When tumor volume, in each group, reached ~100 mm 3 , mice were killed, and tumors were removed and weighed for use in histology and further studies. The tumor volume was calculated using the formula V = 1/2 × larger diameter × (smaller diameter) 2 . For in vivo lung metastasis model, mice were injected with sh-control and sh-METTL3 Huh7 cells, or HeLa WT, Mettl3 Mut/− HeLa, HeLa Snail , and Mettl3 Mut/− HeLa Snail stable cells (1 × 10 6 per mouse, n = 10 for each group). Eight weeks after injection, mice were killed and metastatic lung tumors were analyzed. Immunohistochemistry (IHC) Immunohistochemistry (IHC) was performed to measure expression of target protein according to our previous study [63] . Kaplan–Meier survival analysis and clinical expression analysis Kaplan–Meier plotter ( http://kmplot.com/analysis/ ) is a comprehensive online platform that can assess the effect of 54,675 genes on survival based on 10,293 cancer samples [64] . We used Kaplan–Meier plotter to assess the prognostic value of METTL3, YTHDF1, and SNAI1 expression in patients with liver cancers. mRNA expression of METTL3 and YTHDF1 in cancer tissues and matched adjacent normal tissues of liver cancers were obtained from TCGA (The Cancer Genome Atlas) database. METTL3 expression in HCC tumor tissues ( n = 35), liver cirrhosis tissues ( n = 13) and normal liver tissues ( n = 10) from Oncomine database (Wurmbach liver cancers). mRNA expression of YTHDF1 in liver cancers of T1 ( n = 153), T2 ( n = 77), T3 (n = 65), and T4 ( n = 13) stages from TCGA database. [65] Tissue microarray analysis The protein expression of Mettl3 and Snail in 100 cases of liver cancer patients by use of tissue microarray (CS03–01–008, Alenabio, Xian, Shanxi, China) according to our previous study [66] . The clinical slides of Mettl3 and Snail were analyzed separately by two pathologists without knowing the patients’ clinical information. The intensity was scored on a scale of 0–3 as negative (0), weak (1), medium (2), or strong (3). The extent of the staining, defined as the percentage of positive stained areas of tumor cells per the whole-tumor area, was scored on a scale of 0 (0%), 1 (1–25%), 2 (26–50%), 3 (51–75%), and 4 (76–100%). An overall protein expression score (overall score range, 0– 12) was calculated by multiplying the intensity and positivity scores. For statistical purposes, the staining score was further categorized as low (0–5), medium (6–8), and high (9–12). Statistical analyses Data were reported as mean ± SD from at least three independent experiments unless otherwise specified. Values for capillary tube formation and luciferase activity assays are from three independent experiments that were performed in duplicate. Data were analyzed by two-tailed unpaired Student’s t test between two groups and by one-way ANOVA followed by Bonferroni test for multiple comparison. Statistical analysis was carried out using SPSS 16.0 for Windows. All statistical tests were two sided. A p -value of < 0.05 was considered to be statistically significant. Data are presented as means ± SD from three independent experiments. * p < 0.05, ** p < 0.01. NS, no significant. Reporting summary Further information on research design is available in the Nature Research Reporting Summary linked to this article.